Integrated spatial multiplexing of heralded single-photon sources The non-deterministic nature of photon sources is a key limitation for single-photon quantum processors. Spatial multiplexing overcomes this by enhancing the heralded single-photon yield without enhancing the output noise. Here the intrinsic statistical limit of an individual source is surpassed by spatially multiplexing two monolithic silicon-based correlated photon pair sources in the telecommunications band, demonstrating a 62.4% increase in the heralded single-photon output without an increase in unwanted multipair generation. We further demonstrate the scalability of this scheme by multiplexing photons generated in two waveguides pumped via an integrated coupler with a 63.1% increase in the heralded photon rate. This demonstration paves the way for a scalable architecture for multiplexing many photon sources in a compact integrated platform and achieving efficient two-photon interference, required at the core of optical quantum computing and quantum communication protocols. It has been shown that the quantum nature of single photons could be used to create a quantum computer [1] and to communicate securely [2] . These initial proposals were formulated with the assumption that perfect photon sources would one day exist. Imperfect non-deterministic single-photon sources have limited the complexity of demonstrations to date, despite significant work to simplify quantum operations and ease technical demands [3] . If the single-photon output for multiple indistinguishable sources can be engineered to be more deterministic, this would create a new potential for scalable quantum technology based on photon–photon interference, including boson-sampling processors [4] , [5] , [6] , [7] , long-distance communication [8] and metrology [9] . Several physical systems can be used to generate single photons. Single quantum emitters such as quantum dots [10] , [11] or diamond colour centres [12] potentially offer on-demand single photons, but are difficult to implement on-chip and scale up, owing to challenges in engineering such sources to emit at the same frequency [11] , large-footprint bulk photon collection apparatus and the typical requirement for cryogenics [10] , [11] . Attenuated coherent light sources are frequently used as a source of non-deterministic single photons. They are easy to construct and package, but the output signal-to-noise is fundamentally limited by the Poisson shot noise of a coherent source: a fraction of events will contain more than one photon and the probability of such multiple photons increases with the emission rate. One must inevitably accept either a low photon rate or a significant fraction of multiple photons. A third class, heralded single-photon sources, are based on correlated photon pair generation. By detecting one photon from a pair, the existence and timing of the remaining photon is then known. This additional information is the basis of multiplexing [13] where heralded single photons from multiple sources can be deterministically combined using active switching. Each single source still suffers from multiple events, or multipairs, to essentially the same degree as the attenuated coherent state source. However, now this can be mitigated by using many heralded sources with a lower generation probability, lowering the net rate of multipair generation. In the ideal case of lossless switches, the multipair rate falls in proportion to the number of multiplexed sources. Heralded single-photon sources are often based on photon pairs generated in non-linear optical media, including spontaneous four-wave mixing (SFWM) in χ (3) waveguides [14] , [15] , [16] , [17] , [18] , [19] , [20] and spontaneous parametric down conversion in χ (2) devices [21] , [22] . As stochastic processes, these schemes do display multipair events. If a sufficiently narrow output filter ensures that the generated photons are spectrally indistinguishable, which is usually desirable, the number of photon pairs generated per pulse is governed by thermal photon statistics [23] , [24] , [25] , [26] . For weaker filtering the statistics approach a Poisson limit, as multiple pairs are most likely to be produced in uncorrelated events. Either way, multipair generation introduces noise photons, thus setting a fundamental relationship between the number of photon pairs generated per pulse and the noise performance of the source. Given a mean pair-generation rate per pump pulse of μ , the probability of multiple pairs in a single pulse is P >1 = αμ 2 , where α is of order unity and depends on the filtering [24] . Low-noise photon-pair generation requires sources that operate in a regime of small P >1 . Limiting the mean pair rate μ to be below 0.1 per pulse for instance, allows for a quantum bit error rate below 5% in a quantum communication system [27] . Let us introduce the collection efficiency η as the probability a photon goes through the circuit to the detector. For an integrated device working in the telecommunications wavelengths, η is typically between 10 −2 and 10 −3 because of coupling loss, component loss and imperfect detection. The probability that one photon of a pair is detected per pulse is then μη , meaning that for detecting a heralded single-photon or a two-photon coincidence per pulse, the probability becomes μη 2 . Next, the probability of detecting interference events between the heralded photons from two separate sources is μ 2 η 4 , meaning scalable multiphoton operations are extremely uncommon. As this interference between photons from separate sources is at the core of many quantum gates, the low probability is detrimental to the implementation of many algorithms [28] . Multiplexing many photon pair sources decouples the relationship between the desirable single-photon output and multipair noise governing an individual source, allowing a higher single-pair rate for a fixed multipair (noise) rate. Multiplexing can be implemented with both spatial [13] , [29] , [30] or temporal schemes [31] . The previous demonstration of efficient multiplexing used a free-space scheme [30] , where the use of bulk Mach–Zehnder interferometers made the setup inherently sensitive to alignment stability and used a large amount of space, causing the scalability of such a scheme to be an issue. The advantages of an integrated photonic architecture, in contrast, are that many sources and components can be fabricated onto a single monolithic chip with proven stability [32] . Although this strategy has been highly successful for tunable quantum processing [33] , at present there has been no demonstration for scalable multiplexed single-photon generation. Here we report the experimental demonstration of integrated, spatially multiplexed, heralded single-photon sources. A ceramic optical switch, made from ultra-low loss lead lanthanum zirconium titanate (PLZT) [34] , was used to route photons from two monolithic silicon sources to a common output. We present spatial multiplexing of heralded single photons using the above architecture, for N =2, in two different configurations. The first consists of two photonic crystal waveguides (PhCWs) with the classical pump beam coupled separately to each waveguide on the chip, allowing for ease of balancing the coupled power. The second has, in addition, an on-chip 50:50 Y-coupler to divide the input pump laser between two PhCWs, demonstrating further integration. The setups are all-fibre coupled, stable and robust implementations of spatial multiplexing, making use of integrated optical devices. Our results demonstrate that it is possible to increase the rate of useful single photons by multiplexing together many individual heralded single-photon sources in the telecommunications band using a stable, all-fibre-coupled setup. We achieve 62.4 and 63.1% enhancement to the probability of generating a single photon from a pump pulse without affecting the noise level in two separate experiments, the first on two separately pumped sources and the second with two sources pumped through a common input. These enhancements are limited purely by the insertion loss of the switches. Scaling up to a larger number of devices will facilitate the creation of a new class of useful single-photon sources. 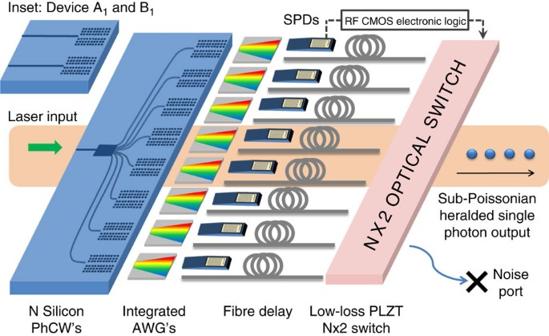Figure 1: Spatial multiplexing scheme. A single laser is coupled to a monolithic silicon chip to pump an ultra-compact array of silicon PhCWs. Photon pairs are generated in the PhCW region, wavelength separated by integrated arrayed waveguide gratings (AWGs) and the heralding photons detected using single photon detectors. The remaining photons go through a delay line, while a fast electronic logic gate sets the state of the PLZT switch. The selected heralded photon is then routed to the common fibre output. The orange box region represents the experimental setup for results presented in this work. Inset: our first implementation used a device with two separate but monolithically fabricated PhCWs, designated A1and B1. Spatial multiplexing scheme Figure 1 shows a schematic of our proposed architecture for efficient spatial multiplexing of N photon pair sources with the aim of building a more deterministic single-photon source. Here the pump pulses are coupled to a silicon waveguide and split to a bank of N nominally identical and monolithically integrated PhCWs, where photon pairs are generated by SFWM, as shown in Fig. 2 . The PhCWs provide strong light confinement, but the major enhancement to the non-linearity is through slow-light engineering [35] —the precise arrangement of the photonic crystal holes induces very strong dispersion so that the pump group velocity c/n g is lower than the value c/n 0 in unpatterned silicon by a factor S = n g /n 0 ≈10. The SFWM process scales as an S 4 enhancement owing to the increase in pump intensity and interaction time, thereby enabling an ultra-compact source [36] . To permit the generation of indistinguishable photon pairs using a single pump laser, the position of the slow-light frequency window must be nominally identical in all PhCWs (see Methods section for more information). The two photons are separated using wavelength division components that can be realized, for example, using integrated arrayed waveguide gratings [37] , [38] . One photon from each pair is detected by an array of N integrated silicon waveguide-based single-photon detectors [39] , whereas the other is buffered in an optical delay line (ODL) [40] , [41] . Currently, this delay line is implemented using optical fibre, as this is the only technology available to provide sufficient delay while remaining at a reasonably low loss. While the photon is delayed, a radio frequency logic gate triggered by a photon detection feeds forward a drive signal to a fibre-coupled opto-ceramic switch, which actively routes single photons to a common output. The switch, which is based on an electro-optic polarization rotation [34] , is fabricated from PLZT and has a maximum switching rate of 1 MHz and an insertion loss of ~1 dB. For a net increase in the heralded photon rate in the case of only two sources, the switch insertion loss must be <3 dB (see ref. 13 ). The output is a multiplexed stream of indistinguishable single photons, given matched post-generation spectral filtering. Figure 1: Spatial multiplexing scheme. A single laser is coupled to a monolithic silicon chip to pump an ultra-compact array of silicon PhCWs. Photon pairs are generated in the PhCW region, wavelength separated by integrated arrayed waveguide gratings (AWGs) and the heralding photons detected using single photon detectors. The remaining photons go through a delay line, while a fast electronic logic gate sets the state of the PLZT switch. The selected heralded photon is then routed to the common fibre output. The orange box region represents the experimental setup for results presented in this work. Inset: our first implementation used a device with two separate but monolithically fabricated PhCWs, designated A 1 and B 1 . 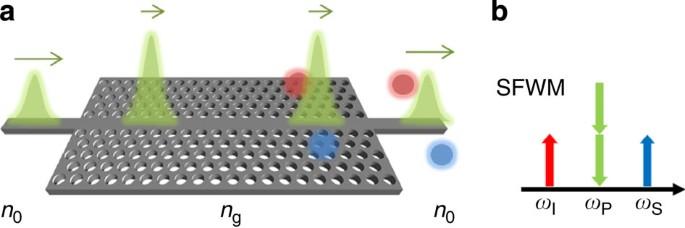Figure 2: Schematic representation of the SFWM process. A pulse of laser light approaches the silicon PhCW shown inaat a speed ofc/n0, wherecis the speed of light andn0is the refractive index of silicon. When the pulse enters the PhCW, it is spatially compressed and travels at a slower speed through the mediumc/ng, wherengis the group index in the PhCW. From this, we define a slow-down factorS=ng/n0. Two photons of the pulse are annihilated to generate signal and idler photons of higher and lower energy, shown as blue and red circles, with the process depicted inb. The process must obey energy and momentum conservation such thatωS+ωI=2ωPandkS+kI=2kP+2γP0, where the subscripts denote signal, idler and pump,γis the non-linear parameter andP0is the peak power in the device. The remaining pulse and photons then exit the PhCW into the fast-light regime. Full size image Figure 2: Schematic representation of the SFWM process. A pulse of laser light approaches the silicon PhCW shown in a at a speed of c/n 0 , where c is the speed of light and n 0 is the refractive index of silicon. When the pulse enters the PhCW, it is spatially compressed and travels at a slower speed through the medium c/n g , where n g is the group index in the PhCW. From this, we define a slow-down factor S = n g /n 0 . Two photons of the pulse are annihilated to generate signal and idler photons of higher and lower energy, shown as blue and red circles, with the process depicted in b . The process must obey energy and momentum conservation such that ω S + ω I =2 ω P and k S + k I =2 k P +2 γP 0 , where the subscripts denote signal, idler and pump, γ is the non-linear parameter and P 0 is the peak power in the device. The remaining pulse and photons then exit the PhCW into the fast-light regime. Full size image Dual-input waveguide device In the first demonstration, the two waveguides are labelled A 1 and B 1 , and are sketched in the inset of Fig. 1 . The rate of pairs from each source was measured before the electro-optic switch and compared with the multiplexed rate measured at the common output. The standard signal-to-noise metric for probabilistic photon-pair sources is the coincidence-to-accidental ratio (CAR). 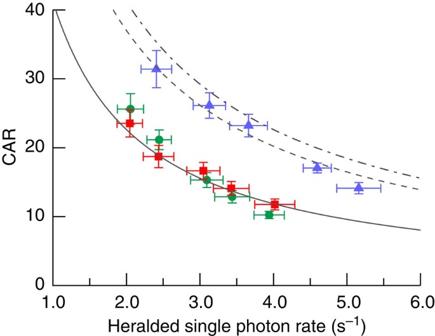Figure 3: Spatial multiplexing result. The CAR from source A1(green circles), source B1(red squares) and after multiplexing (blue triangles) are plotted for a range of heralded single-photon rates. The solid line represents a fit to the single source data, the dashed line represents a fit to the multiplexed data and the dot-dashed line represents the expected enhancement for a lossless switch. All errors are calculated from Poissonian statistics. Figure 3 illustrates the CAR for a range of measured heralded single-photon rates for individual PhCWs A 1 and B 1 , shown as red squares and green circles, respectively. The characteristic curve for the measured CAR of an individual source is limited by multipair noise. The absolute rate was then estimated by taking into account component losses and detector efficiencies. We spatially multiplexed the two sources by adding in an optical switch and electronics to route photons to a common output fibre. The multiplexing measurements were made using the same characterization setup as for the individual sources and the result is plotted in Fig. 3 as blue triangles. We fitted the data for the single sources using an analytical expression for the CAR ratio, including the measured values for detector dark counts and losses (see Methods section). By measuring the transmission of the opto-ceramic switch channels (85.1 and 79.4%), we calculated the maximum expected enhancement to the CAR as a function of the heralded single-photon rate (dashed line in Fig. 3 and see Supplementary Fig. S1 for more detail). It can be seen that the data is entirely consistent with this maximum expected enhancement and that the results for the multiplexing case lie well above the limit for a single source of this type. Indeed, to check the agreement we fit the data to the predicted curve, but allowing the switch transmission to vary. The best fit was obtained for a transmission that slightly exceeds the measured values, so that within experimental error we have obtained the maximum possible performance. We also show the theoretical case for a lossless switch and note that we are operating close to this regime. For a fixed CAR, we achieved a 62.4% improvement in the detected single-photon rate, equivalent to increasing the probability of generating a photon, while maintaining a constant probability of multipair noise. Similarly, an improvement in the CAR was achieved for a fixed photon rate, which corresponds to a reduction in the multiphoton noise. The decoupling of the single-photon and multiphoton rates, evident in the result shown in Fig. 3 , is the essence of spatial multiplexing. To provide a clear demonstration, the measurement was made in the regime where multiphoton generation is the dominant noise source, at rates well above the dark-count-limited CAR peak [18] . Note that other methods to enhance the single-photon rate, including increasing pump power or pump-laser repetition rate [42] , cannot be used to achieve the same decoupling and the noise level scales as for individual sources. Figure 3: Spatial multiplexing result. The CAR from source A 1 (green circles), source B 1 (red squares) and after multiplexing (blue triangles) are plotted for a range of heralded single-photon rates. The solid line represents a fit to the single source data, the dashed line represents a fit to the multiplexed data and the dot-dashed line represents the expected enhancement for a lossless switch. All errors are calculated from Poissonian statistics. Full size image Single-input waveguide device The second experimental implementation demonstrates a primary building block for our proposed scheme and is shown schematically as the region inside the orange box in Fig. 1 . The two PhCW devices are referred to as A 2 and B 2 , shown in the scanning electron micrograph, Fig. 4a . The output heralded single-photon rate from each waveguide was measured and plotted in Fig. 4b , shown as green triangles and red squares for A 2 and B 2 , respectively. The multiplexing switch was then added and the multiplexed output measured for the same range of PhCW output powers, shown in Fig. 4b as blue triangles. We extract an enhancement to the heralded single-photon rate of 63.1% (see Methods section and Supplementary Fig. S2 ), consistent with the result of the first measurement. 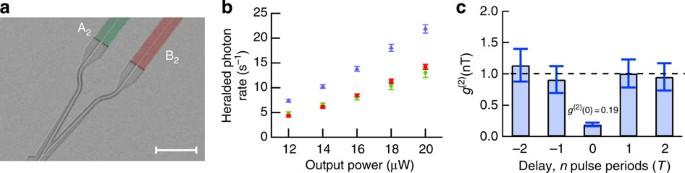Figure 4: On-chip Y-split coupler. (a) A scanning electron microscope image of an integrated waveguide-based Y-split geometry 50/50 coupler, splitting incoming pump pulses between two PhCWs A2and B2shown in green and red false colour, respectively. Scale bar, 20 μm. (b) Heralded single-photon rates from source A2(green circles), source B2(red squares) and the multiplexed (blue triangles) rate are plotted for a range of output powers. (c) Theg(2)(nT) correlation function is measured for the multiplexed output, a value ofg(2)(0)=0.19, markedly <0.5, confirms the source is operating in the single-photon regime. For other values ofn, the uncorrelated Poissoniang(2)(nT) is close to 1, as shown by the dashed line. All errors are calculated from Poissonian statistics. Figure 4: On-chip Y-split coupler. ( a ) A scanning electron microscope image of an integrated waveguide-based Y-split geometry 50/50 coupler, splitting incoming pump pulses between two PhCWs A 2 and B 2 shown in green and red false colour, respectively. Scale bar, 20 μm. ( b ) Heralded single-photon rates from source A 2 (green circles), source B 2 (red squares) and the multiplexed (blue triangles) rate are plotted for a range of output powers. ( c ) The g (2) ( nT ) correlation function is measured for the multiplexed output, a value of g (2) (0)=0.19, markedly <0.5, confirms the source is operating in the single-photon regime. For other values of n , the uncorrelated Poissonian g (2) ( nT ) is close to 1, as shown by the dashed line. All errors are calculated from Poissonian statistics. Full size image Second-order correlation function measurements To verify that the output of our multiplexed source was indeed in the single-photon regime, we measured the second-order correlation function g (2) ( nT )= C ABH C H /C AH C BH at discrete delays using a Hanbury–Brown and Twiss (HBT) setup [43] , [44] . Here, C ABH is a threefold coincidence across all detectors, C AH and C BH are the heralded clicks in detectors A and B, C H is the number of heralding clicks, n is an integer and T is the period between pump-laser pulses. A measured g (2) (0)<1 is expected for a non-classical light source and g (2) (0)<0.5 for a source approaching true single-photon operation. A 50/50 coupler is required for an HBT experiment, and was added to the common output. An ODL was added to adjust the fine balance in optical path length (see Methods section), with the requirement that the optical paths from each of the photon-pair sources and the coupler be balanced. In this experiment, sources A 2 and B 2 both contribute to the measured photon statistics used to calculate g (2) ( nT ), which is plotted in Fig. 4c . The measured g (2) (0)=0.19±0.02 confirms that our spatially multiplexed source is operating in the single-photon regime. As a check of this result, we measured g (2) ( nT ) for n =±1,2, delaying or advancing the electronic trigger pulses from the detector at one output of the 50/50 coupler by one or two pulse periods with respect to the other and measuring the correlation. For these correlations between successive pulses, we expect the photon statistics to return to a Poissonian distribution with g (2) (± nT )=1. The measured g (2) (+ T )=1.01±0.23, g (2) (− T )=0.91±0.21, g (2) (−2 T )=1.14±0.26 and g (2) (+2 T )=0.95±0.22 are consistent with this expectation. The N x2 switch indicated in Fig. 1 can be accomplished with the technology described here by a series of cascaded switches. For low dark counts and low single-channel pair rates μ , the expected net enhancement with N sources is , where the switch transmission is η L . If we were to extend this demonstration using multiple PLZT switches with 1 dB loss each, for example, scaling to eight sources requiring the realistically achievable number of nine detectors and seven switches, this would provide an enhancement of the heralded single-photon rate by a factor of four [45] , [46] . This corresponds to a >16-fold increase in the two-photon interference events between separate sources required for the operation of, for example, a quantum relay [47] or a controlled NOT gate [32] , [48] . PhCWs are ideal sources for this scheme because of their broadband slow-light enhancement that enables compact device design even with a spectrally broad pulsed pump. The efficiency of the heralding detectors used here were limited to 10% when operating at 1,550 nm with reasonable dark-count levels. The combination of this detector inefficiency and coupling losses from the PhCWs caused a low heralding efficiency in this experiment of ~1%. In a multiplexed source, any improvement to the detector or heralding efficiency carries over favourably to the single-photon output rate. For example, doubling the detection efficiency for a source with N multiplexed waveguides would result in a 2 N increase in the heralded single-photon rate. The linear losses associated with the waveguide and filtering components will likely be reduced in step with advances in fabrication technology, further increasing the single-photon rate. Other integrated optical switching technology, such as thermal switching in silicon devices and electro-optic effects in lithium niobate Mach–Zehnder interferometer arrays, may yet prove to be preferable technology when scaling to large numbers of switches, as one would only be penalized with one input and output insertion loss for the whole array. Although the current demonstration of spatial multiplexing implemented here is not monolithically integrated onto a single-photonic chip, it is all-fibre coupled, making it a stable and robust platform for increasing the determinacy of heralded photon sources. A major hurdle in moving to a monolithic device is the development of low-loss ODLs that are compatible with low-noise photon pair sources, preferably in a single-material platform, which is currently not the case. We are aware that recent integrated sources show superior output photon statistics, including heralding efficiencies, to those presented here [20] , but stress the fact that this multiplexing scheme is applicable to any of these sources and will give a comparable improvement to the heralded photon rate at a constant signal-to-noise. This demonstration provides a road map for the creation of fully integrated near-deterministic heralded single-photon sources. Our results show that integrated spatial multiplexing can be implemented efficiently to overcome the non-deterministic nature of single-photon sources currently limiting applications requiring many single photons. We achieved an enhancement to the probability of generating a single photon of 62.4 and 63.1%, breaking the intrinsic limit of a single source by decoupling the single and multipair noise probabilities. Our building-block demonstration establishes the feasibility of scalable multiplexed sources, which promise a new domain of fundamental investigations in quantum mechanics, including high-photon number entanglement, complex quantum computation schemes and highly efficient quantum communication. Multiplexing will continually benefit from technological development in the areas of ultrahigh efficiency detectors, low-loss integrated optics and precision fabrication, leading to more impressive multiqubit (>10) demonstrations using a stable source. Device fabrication The silicon PhCWs were fabricated from a silicon-on-insulator wafer, with a 220-nm-thick Si layer above a 2-μm layer of silica. The photonic crystal was patterned using electron beam lithography and reactive ion etching to create a triangular lattice of holes. The waveguides were made by introducing a row defect. The photonic crystal region was then undercut, by etching away the silica substrate in that region, suspending the PhCWs in air. The two rows of holes adjacent to the waveguide were laterally shifted to engineer the dispersion [35] such that the group index was ~30 across an ~15-nm bandwidth and centred at a wavelength of 1,559 nm. The effective non-linearity ( γ eff =( n g / n 0 ) γ ) was ~4,000 W −1 m −1 , where the slow-down factor S and the ratio of the group index n g to the native refractive index of the material n 0 is included. The PhCW had a linear propagation loss of ~50 dB cm −1 . The waveguides were 196-μm long, with inverse tapers and SU8 polymer cladding for improved coupling by mode matching to input–output lensed fibres. The first device measured had many separate PhCWs with individual input and output coupling. The second sample included Y-split couplers, fabricated using silicon nanowires preceding the pairs of PhCWs. The PhCW regions were fabricated as close as possible to each other, to avoid variations in the Si layer thickness across the surface of the wafer, minimizing any differences in the dispersion and group index. Experimental methods for spatial multiplexing In the first experiment, ~7-ps laser pulses were separated off-chip with a 50:50 fibre-based directional coupler and coupled to on-chip polymer access waveguides using a lensed fibre. For the second experiment, a Y-split coupler was integrated on to the same chip as the PhCWs and the pump coupled to the device via a single lensed fibre and input polymer waveguide. The pulses were thus divided and then coupled into the two PhCWs, which had nominally identical dispersion properties and slow-down factors, S ≈10. In the PhCW regions, correlated photon pairs were generated via SFWM, whereby two photons from the pump pulse are annihilated to generate signal and idler photons of higher and lower energy, respectively, which must obey both energy- and phase-matching conditions, shown schematically in Fig. 2 . The efficiency of generating photon pairs was enhanced by the slow-light effects in the PhCWs [49] , where there is a simultaneous enhancement to the peak power in the device as the light slows down and a longer interaction time as the slowed pulse propagates through the non-linear medium. Care must be taken to not operate in a regime of enhanced non-linear loss [50] . Each pair was coupled out of the device, again using inverse tapers and lensed fibres to minimize loss. The photons from each pair were separated into two single-mode optical fibres using a pair of arrayed waveguide gratings with a photon-channel detuning of 300 GHz from the pump channel. The signal photons were detected using superconducting single-photon detectors (SSPDs). The SSPDs, with a maximum allowed count rate of ~10 MHz, were operated at ~10% efficiency with dark counts of ~100 s −1 and integration times ranged from 5 to 15 min for the highest and lowest powers, respectively. These detection events provided the heralding electrical pulses that triggered the optical switch. Depending on whether source A or B generated a pair, the optically transparent ceramic switch [34] routed the remaining idler photon from each pair to the common output fibre where they were detected using a third SSPD. All counts were then analysed for coincident detection using a time-interval analyser and measured as a histogram (see Supplementary Table S1 for tabulated results). Coincidence counts were taken in a histogram with respect to the delay time. Coincidences at zero time delay include the desired contribution from single pairs, but also from noise components, including detector dark counts, unsuppressed pump photons, uncorrelated spontaneous Raman scattering in any silica components and multipair generation, collectively known as accidental counts. The accidental counts and genuine counts, which arise in the same pulse, cannot be deterministically separated; thus, one characterizes the accidental counts by measuring subsequent pulse correlations with the original. Extracting the multiplexing enhancement To calculate the enhancement to the two separately pumped PhCWs, we modelled a single source and the multiplexed source, including the switch efficiencies. We start by taking a single source, noting that true coincidences C (1) per pulse generated through SFWM can be expressed as C (1) = μη S η I , where μ is the number of pairs generated per pulse, and η S and η I are the overall collection efficiencies for the signal and idler photons, respectively. Here we use a lump statistics approach and ensure μ <0.1. The accidentals can then be calculated as the product of the singles rates N S,I = μη S,I + d S,I , such that A (1) = N S N I =( μη S + d S )( μη I + d I ), where d S and d I are the dark counts in the signal and idler detectors, respectively. We calculate CAR (1) by taking the ratio of coincidences to accidentals such that We can substitute μ = C (1) / η S η I in the denominator to obtain an equation that is only dependent on C (1) For the two source multiplexed case, we can express the coincidences at the output of the switch as C (2) = μη S η I η L1 +(1− μη I − d I ) μη S η I η L2 , whereas the accidentals are A (2) = A 1 (2) + A 2 (2) =( μη I + d I )( μη S η L1 + d S )+(1− μη I − d I ) × ( μη I + d I )( μη S η L2 + d S ). Here, η L1,L2 are the switch losses for the two sources, and we have assumed that the detector dark counts and idler efficiencies are balanced for the two sources. We can then substitute for μ as in the single-source example and obtain an expression for the enhanced CAR (2) for two sources in terms of C (1) Using these equations, we can create a parametric plot of CAR versus C (1) R , where R is the repetition rate of the laser and can compare this with our experimental data, shown in Supplementary Fig. S1 . To calculate η S,I , we take single-source measurement data, plotted as green circles and red squares, which we then fit using equation (2) with our measured dark counts per pulse d S = d I =2 × 10 −6 and take the average, shown as a red dashed line resulting in η S = η I =0.001. We then use these parameters in equation (3) and take the experimentally measured switch losses of η L1 =0.79 and η L2 =0.85 to plot the multiplexed curve shown as a blue solid line, which is in agreement with the data shown as blue triangles. We also show the case for a lossless switch ( η L1 = η L2 =1) as a black dotted curve. We can then numerically extract the experimental enhancement by taking the ratio of the multiplexed count output C (2) and the single-source rate C (1) , which when calculated is 62.4%. To fit the data of coincidences versus power for the Y-split device, we used a similar method. We take the equation to describe coincidences per second C (1) = μη S η I R and the fact that μ = A ( γ PL ) 2 , where P is the coupled power, γ is the non-linear parameter, L is the length of the waveguide and A is a constant that is dependent on the efficiency of the SFWM process and any coupling of the power to the waveguide. We then plot the single source data, shown as green circles and red squares in Supplementary Fig. S2 , and fit these curves before finding an average fit, shown as the red dashed line, to find RA ( γL ) 2 η S η I . We can then again write the multiplexed output as C (2) = Rμη S η I η L1 + R (1− μη I ) μη S η I η L2 , and insert RA ( γL ) 2 η S η I and the measured switch losses of η L1 =0.79 and η L2 =0.85 to plot the multiplexed curve shown as a blue solid line, which is in agreement with the data shown as blue triangles. The enhancement is then simply the ratio of these curves, which gives an enhancement of 63.1%. We again show the case for a lossless switch with an enhancement of 100% as a black dotted curve. Measuring the second-order correlation function We measured the second-order correlation function g (2) ( nT ) after multiplexing the photons from two PhCWs using an HBT setup. The setup was modified by adding a 50:50 directional coupler to the common output and a fourth detector, noting n is an integer and T is the time between each successive pump pulse; together, nT is the difference in arrival time to the detector between photons exiting the two outputs of the coupler. At zero time delay between the detectors, a g (2) (0)<1 is expected for a non-classical light source and g (2) (0)<0.5 for a source approaching single-photon operation. The measured g (2) (0)=0.19±0.02 confirms that the spatially multiplexed source is operating in the single-photon regime. We verified the validity of our measurement by determining g (2) (±1T, ±2T) for neighbouring pulses, which were found to be unity within error, consistent with the Poissonian statistics expected when measuring distinguishable photons [17] , [18] , [48] . The data for all five peaks were taken for 7 h each, resulting in a total number of threefold counts for the g (2) (0) case of 46, and 18–20 counts for all other cases. See Supplementary Table S2 for tabulated results. How to cite this article: Collins, M. J. et al. Integrated spatial multiplexing of heralded single-photon sources. Nat. Commun. 4:2582 doi: 10.1038/ncomms3582 (2013).